Self-assembly and modular functionalization of three-dimensional crystals from oppositely charged proteins Multicomponent crystals and nanoparticle superlattices are a powerful approach to integrate different materials into ordered nanostructures. Well-developed, especially DNA-based, methods for their preparation exist, yet most techniques concentrate on molecular and synthetic nanoparticle systems in non-biocompatible environment. Here we describe the self-assembly and characterization of binary solids that consist of crystalline arrays of native biomacromolecules. We electrostatically assembled cowpea chlorotic mottle virus particles and avidin proteins into heterogeneous crystals, where the virus particles adopt a non-close-packed body-centred cubic arrangement held together by avidin. Importantly, the whole preparation process takes place at room temperature in a mild aqueous medium allowing the processing of delicate biological building blocks into ordered structures with lattice constants in the nanometre range. Furthermore, the use of avidin–biotin interaction allows highly selective pre- or post-functionalization of the protein crystals in a modular way with different types of functional units, such as fluorescent dyes, enzymes and plasmonic nanoparticles. Ordered molecular clusters [1] , nanoparticle superlattices [2] and colloidal crystals [3] have been extensively pursued in order to develop hierarchically structured nanomaterials with tuneable optical, magnetic, electronic and catalytic properties [4] , [5] . Binary and ternary crystals have received focused attention because they provide an approach to integrate different components to yield multifunctional metamaterials, where new properties arise from collective behaviour [6] , [7] . Such nanomaterials are important for applications, but can also provide a fundamental understanding to aid the constructions of different superlattice structures [8] , [9] , [10] . Besides using alkanethiolate-stabilized nanoparticles, binary nanoparticle superlattices with programmed structural diversity can also be prepared from functionalized nanoparticles, for example, through electrostatic interactions [11] , [12] . Recent development in DNA engineered superlattices has considerably extended the range of possible nanoparticle arrangements and types [13] , therefore allowing tailored colloidal crystal structures and lattice parameters [14] , [15] , [16] . Most of the superlattice structures rely fully or partly on synthetic particles, and the use of native biomolecules has consequently remained elusive. However, some important biohybrid structures have been recently presented [17] , [18] . For example, small tetragonal two-dimensional (2D) arrays were prepared from genetically histidine-tagged proteins and gold nanoparticles (AuNPs) interconnecting the tag sites [19] . An extension to three-dimensional (3D) structures was achieved by using electrostatic self-assembly of AuNPs and protein cages, such as ferritins and virus particles, to create binary crystals [20] . In addition, DNA-mediated assembly has yielded binary crystal with NaTl lattice [21] . Also programmable protein-based lattices have been recently introduced [22] , [23] , [24] , [25] , [26] , [27] . For example, Crysalin technology has presented the formation of protein lattices through the genetic fusions between oligomeric proteins with matching rotational symmetry [23] . Such assemblies can be used as sensors or to orient and attach guest molecules to aid their structural characterization with electron microscopy or X-ray scattering [28] . Superlattices with many different nanoparticle arrangements can be achieved through these approaches; however, preparation of truly 3D heterogeneous crystals, especially without the help of DNA, has proved to be a challenging task [23] , [29] . Although binary crystals have been assembled from synthetic and biological building blocks, the combination of different protein-based building blocks into a single binary crystal is not trivial and has consequently remained underexploited. Such binary protein crystals would, however, allow the preparation of biologically active systems in polar aqueous media differing from entropy driven hard sphere assemblies and emulate complex protein assemblies found in nature. Furthermore, a broadly applicable system for modular functionalization of the crystal structures is required for advanced biomedical applications. Here we present a conceptually new strategy to self-assemble binary crystals from biological building blocks, namely two different proteins with opposite net charges that are presented in patches on the protein surface. We combine oppositely charged cowpea chlorotic mottle virus (CCMV) particles (isoelectric point (pI) ~3.8) and avidin (pI ~10.5) into binary crystals by using electrostatic interactions, which allows crystal formation without covalent modification of the protein cages and make the crystals responsive to external stimuli, such as pH and electrolyte concentration. Furthermore, the use of avidin allows straightforward modular functionalization of the nanostructures through the well-known avidin–biotin technology. We show that the crystals can be pre- or post-functionalized with various biotin-tagged building blocks, including fluorescent dyes, enzymes and AuNPs. Protein-based materials Biological building blocks, such as protein cages (for example, CCMV and ferritins) and avidin ( Fig. 1 ), are widely used in nanotechnology and biotechnological applications [30] , [31] . Protein cages can effectively constrain and template the formation of nanoparticles [32] , [33] . Owing to their highly monodisperse structure, protein cages also readily form ordered arrays on solid supports or interfaces [34] , [35] . Furthermore, we have shown that protein cages can form free-standing crystals or crystalline assemblies in solution with the help of synthetic binding agents [36] , [37] , [38] . CCMV consists of 180 identical coat protein subunits that encapsulate the RNA genome to yield a T =3 viral particle ~28 nm in diameter, which exhibits large negatively charged patches around the 60 pores present in the centre of the threefold quasi-icosahedral rotation axes ( Fig. 1a ). On the other hand, avidin is a tetrameric glycoprotein ( M w 68 kDa) that binds biotin with extreme selectivity and affinity. This ability has allowed avidin and its derivatives to become an important tool in many biochemical techniques, including biomolecule detection, interaction studies and purification. Avidin has a maximum cross-section of 7.2 nm and hydrodynamic diameter of 5.4 nm measured by dynamic light scattering (DLS; Fig. 1b ). The four positively charged patches are arranged in tetrahedral geometry. The characteristics of the patchy electrostatic potential map of avidin can be described as a rigid tetrahedron with four positive patches in the corner points of the tetrahedron ~5.1 nm apart. Examples from previous studies show that a patchy interaction pattern strongly affects the final structure of self-assembled nanostructures [39] , [40] , [41] , [42] , [43] . Also, the geometrical shape has been shown to guide the self-assembly of non-spherical particles [44] , [45] , [46] . 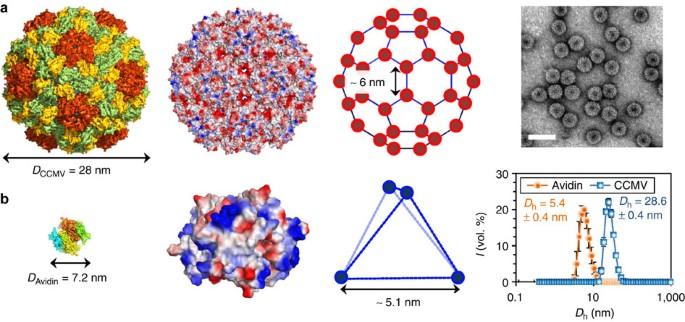Figure 1: Protein-based materials used to form electrostatic binary solids. (a) Native CCMV and (b) avidin. From left to right: particles drawn to scale, calculated electrostatic surface potential, location and geometry of patches, TEM image of negatively stained CCMV (scale bar, 50 nm) and DLS measurements of avidin and CCMV (volume-weighted size distribution). Figure 1: Protein-based materials used to form electrostatic binary solids. ( a ) Native CCMV and ( b ) avidin. From left to right: particles drawn to scale, calculated electrostatic surface potential, location and geometry of patches, TEM image of negatively stained CCMV (scale bar, 50 nm) and DLS measurements of avidin and CCMV (volume-weighted size distribution). Full size image Self-assembly of CCMV–avidin crystals Electrophoretic mobility, DLS and small-angle X-ray scattering (SAXS) experiments were first used to study the electrostatic binding between CCMV and avidin leading to the formation of large self-assembled protein crystals ( Fig. 2 ). Gel electrophoresis mobility shift assay indicates that without avidin, the CCMV particles are free, negatively charged and consequently show a high electrophoretic mobility towards the cathode. When avidin/CCMV w / w ratio is increased, CCMV particles gradually lose their mobility, and at a ratio of 0.64 most of the virus particles are bound into larger complexes with very low electrophoretic mobility ( Fig. 2a ). The electrophoretic mobilities were further quantified with laser Doppler velocimetry. CCMV particles in a solution containing no or very small amounts of avidin were measured to have mobilities between −1.5 × 10 −4 and −1.2 × 10 −4 cm 2 V −1 s −1 . At an avidin/CCMV mass ratio between 0.16 and 0.32, the electrophoretic mobility shifts from negative to positive reaching a final value of 1.6 × 10 −4 cm 2 V −1 s −1 at an avidin/CCMV mass ratio of ~0.64 ( Fig. 2b ). Solvated ions screen the electric field of charged particles that makes the CCMV–avidin assemblies sensitive to variations in the ionic strength of the solution. DLS experiments showed that large CCMV–avidin complexes ( D h >1 μm) are formed at low ionic strength. However, they are rapidly disassembled when c NaCl is increased to ~50 mM ( Fig. 2c,d ). The disassembly of CCMV–avidin complexes due to increasing ionic strength is a reversible process, and the structures can reassemble when the ionic strength is decreased. The complex formation is rapid in all cases and takes place within minutes ( Supplementary Fig. 1 ). 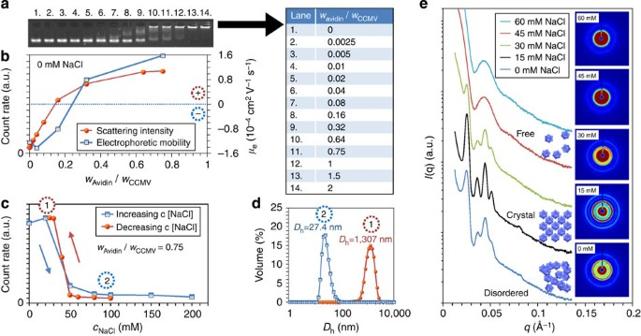Figure 2: Aqueous electrostatic self-assembly of binary CCMV–avidin crystals. Agarose gel electrophoresis mobility shift assay (a), electrophoretic mobility (μe) and dynamic light scattering (b) show the formation of large assemblies, which can be disassembled or reassembled by increasing (to 50 mM NaCl) or decreasing the electrolyte concentration, respectively (c). a.u., arbitrary units. Count rate in decreasingcNaClcurve is multiplied by 0.72 for clarity. Volume-average size distribution measured from the free proteins and binary assemblies (d). Integrated SAXS curves (vertically offset for clarity) show the evolution of scattering curves at different electrolyte concentrations (e). The longest correlation length is achieved at 15 mM NaCl concentration, which is the optimum for crystal formation. Figure 2: Aqueous electrostatic self-assembly of binary CCMV–avidin crystals. Agarose gel electrophoresis mobility shift assay ( a ), electrophoretic mobility ( μ e ) and dynamic light scattering ( b ) show the formation of large assemblies, which can be disassembled or reassembled by increasing (to 50 mM NaCl) or decreasing the electrolyte concentration, respectively ( c ). a.u., arbitrary units. Count rate in decreasing c NaCl curve is multiplied by 0.72 for clarity. Volume-average size distribution measured from the free proteins and binary assemblies ( d ). Integrated SAXS curves (vertically offset for clarity) show the evolution of scattering curves at different electrolyte concentrations ( e ). The longest correlation length is achieved at 15 mM NaCl concentration, which is the optimum for crystal formation. Full size image The crystallinity of aqueous CCMV–avidin complexes at different electrolyte concentrations was probed with SAXS ( Fig. 2e ). In the absence of added electrolyte, electrostatic interactions dominate the complex formation and the assembly process yields kinetically trapped disordered aggregates. However, when c NaCl is increased to 15 mM the strength of electrostatic interactions is reduced, allowing the system to self-assemble into energetically favoured crystals. When the electrolyte concentration is further increased, the correlation length is observed to decrease, as the crystals start to break apart. At even higher electrolyte concentrations ( c NaCl ≥45 mM), only a scattering curve corresponding to the form factor of virus particles is observed ( Supplementary Fig. 2 ), indicating the presence of free particles. This observation is in excellent agreement with the DLS data, and in essence follows the well-characterized behaviour of complex coacervates [47] , [48] , [49] . Nanostructure of self-assembled crystals Integrated scattering curve measured from aqueous suspension of CCMV–avidin crystals in the presence of 15 mM NaCl shows multiple clear diffraction maxima indicating long range order prevalent in the assemblies ( Fig. 3a ). The 2D diffraction patterns show multiple Debye rings typical to polycrystalline samples with isotropic orientation of multiple crystals as in powder-like samples ( Fig. 3b ). The positions of the diffraction peaks in the azimuthally integrated curve are found at q =0.025, 0.036, 0.044, 0.051 and 0.057 Å −1 corresponding to the crystal plane reflections with Miller indices ( hkl )=(110), (200), (211), (220) and (310), respectively. The q n / q * ratio follows ✓ 2: ✓ 4: ✓ 6: ✓ 8: ✓ 10, indicating a cubic lattice. The quadratic Miller indices were plotted against the measured q (hkl) values and fitted with linear regression to obtain the lattice constant a . For cubic phases a saxs =2 π ✓ ( h 2 + k 2 + l 2 )/ q (hkl) , which was determined to be 35.0 nm ( Fig. 3c ). Based on the positions, widths and the relative intensities of the diffraction maxima, the structure is best described as finite body-centred cubic (bcc) Bravais lattice structure (space group , number 229; Fig. 3d ). The crystal structure of CCMV–avidin assemblies obtained from SAXS studies was further verified by cryogenic transmission electron microscopy (cryo-TEM) that supported the bcc crystallographic arrangement. The crystals identified in standard and low-magnification ( Supplementary Fig. 3 ) images were 3D polycrystallites with single-crystal-domain sizes approaching 1 μm ( Fig. 3e ). An image featuring a crystal viewed along the [100] projection axis shows the expected cubic arrangement (unit cell highlighted in cyan) with a measured lattice constant a TEM =35.9 nm ( Fig. 3f–h ). 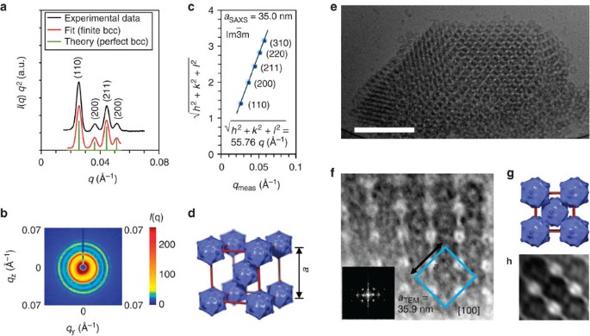Figure 3: SAXS and cryo-TEM characterization of binary CCMV–avidin crystals. (a) Integrated and indexed SAXS curve measured from self-assembled CCMV–avidin crystals and comparison with calculated curves. (b) 2D scattering pattern. (c) Quadratic Miller indices of assigned reflections forstructure versus measuredq-vector positions for five indexed peaks. Solid line presents a linear fit, which yields a lattice parameteraSAXS=35.0 nm (for cubic phasesa=2π✓(h2+k2+l2)/q(hkl)). (d) CCMV–avidin crystal adopts a bcc arrangement (particle size reduced for clarity). (e) Low-magnification view of CCMV–avidin binary crystal in random orientation. Scale bar, 200 nm. (f) Crystal viewed along the [100] projection axis. One unit cell with measuredaTEM=35.9 nm is outlined with cyan. Inset shows a fast Fourier transform image. (g) A model unit cell viewed along [100] projection axis. (h) Filtered inverse Fourier transform from selected Fourier components. Figure 3: SAXS and cryo-TEM characterization of binary CCMV–avidin crystals. ( a ) Integrated and indexed SAXS curve measured from self-assembled CCMV–avidin crystals and comparison with calculated curves. ( b ) 2D scattering pattern. ( c ) Quadratic Miller indices of assigned reflections for structure versus measured q -vector positions for five indexed peaks. Solid line presents a linear fit, which yields a lattice parameter a SAXS =35.0 nm (for cubic phases a =2 π ✓ ( h 2 + k 2 + l 2 )/ q (hkl) ). ( d ) CCMV–avidin crystal adopts a bcc arrangement (particle size reduced for clarity). ( e ) Low-magnification view of CCMV–avidin binary crystal in random orientation. Scale bar, 200 nm. ( f ) Crystal viewed along the [100] projection axis. One unit cell with measured a TEM =35.9 nm is outlined with cyan. Inset shows a fast Fourier transform image. ( g ) A model unit cell viewed along [100] projection axis. ( h ) Filtered inverse Fourier transform from selected Fourier components. Full size image Assuming a spherical 28 nm diameter CCMV particle, a close-packed bcc structure would have a unit cell size of 32.3 nm. According to SAXS, the unit cell size of the final bcc structure of CCMV–avidin complex is 35.0 nm. In this unit cell, the smallest centre-to-centre distance between CCMV particles is d CCMV–CCMV = a ✓ 3/2=30.3 nm leaving an ~2.3 nm spacing between adjacent CCMV particles (for example, between CCMV particles in positions (0,0,0) and (0.5,0.5,0.5) in the unit cell). The bcc structure includes both tetrahedral and octahedral voids when CCMV is located in the lattice points of the unit cell. The tetrahedral voids in this unit cell have a diameter of 11.1 nm and the octahedral voids have a diameter of 7.0 nm. Values indicate that avidin can occupy both the tetrahedral and the octahedral voids. Avidin has to be located mainly in the edge of the voids to allow electrostatic bridging between the CCMV particles since the voids are too large for one avidin alone to fill and the space between two adjacent CCMV particles is too narrow to host even one avidin. Furthermore, the tetrahedral orientation of the positive patches of avidin can optimize their interaction with CCMV when located in the tetrahedral void. The CCMV particles do not form a close-packed structure and the voids are overlapping, which indicates that avidin can still form a continuous matrix around the CCMV particles. Based on the SAXS data and cryo-TEM images ( Fig. 3 ), we argue that CCMV occupies the lattice points of the bcc structure, and the avidin proteins are distributed within the corners of tetrahedral and octahedral inter-particle voids in the lattice to yield a AB 12 bcc structure ( Fig. 4 , and the Supplementary Discussion ). Such a crystallographic arrangement has previously been observed for instance with bcc-packed γ -cyclodextrin 6 cubes held together by potassium ions [50] . 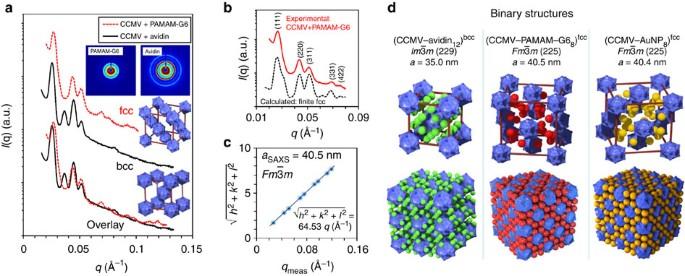Figure 4: Comparison of CCMV crystals formed with avidin and PAMAM-G6. (a) 2D scattering patterns and azimuthally integrated curves show that patchy avidin particles direct the formation of an open bcc CCMV-lattice, whereas isotropically charged PAMAM-G6 forms fcc crystal lattices with CCMV. Top two curves are vertically offset for clarity. (b) Integrated and indexed SAXS curve measured from self-assembled CCMV–PAMAM-G6 crystal and comparison with a calculated finite fcc structure using a core-shell model. (c) Quadratic Miller indices of assigned reflections forstructure versus measuredq-vector positions. Nine peaks can be indexed to the given structure. Solid line presents a linear fit, which yields a lattice parameteraSAXS=40.5 nm. (d) Crystallographic arrangement and lattice parameter details of suggested binary structures of CCMV–avidin, CCMV–PAMAM-G6 and comparison with our previously reported CCMV–AuNP AB8fcc-type lattice20. Figure 4: Comparison of CCMV crystals formed with avidin and PAMAM-G6. ( a ) 2D scattering patterns and azimuthally integrated curves show that patchy avidin particles direct the formation of an open bcc CCMV-lattice, whereas isotropically charged PAMAM-G6 forms fcc crystal lattices with CCMV. Top two curves are vertically offset for clarity. ( b ) Integrated and indexed SAXS curve measured from self-assembled CCMV–PAMAM-G6 crystal and comparison with a calculated finite fcc structure using a core-shell model. ( c ) Quadratic Miller indices of assigned reflections for structure versus measured q -vector positions. Nine peaks can be indexed to the given structure. Solid line presents a linear fit, which yields a lattice parameter a SAXS =40.5 nm. ( d ) Crystallographic arrangement and lattice parameter details of suggested binary structures of CCMV–avidin, CCMV–PAMAM-G6 and comparison with our previously reported CCMV–AuNP AB 8 fcc -type lattice [20] . Full size image In order to demonstrate that the open bcc structure in CCMV–avidin crystals is directed by patchy interactions and is not an effect of the size ratio of the two components, avidin was substituted to an amine-terminated generation six poly(amidoamine) dendrimer (PAMAM-G6). PAMAM-G6 is a sequentially branched polymer with a diameter of ~6.5 nm and molecular weight of 58 kDa. Contrary to avidin, the cationic surface of PAMAM-G6 is not patchy and the object can be viewed as a globular smoothly charged nanoparticle. Hence, PAMAM-G6 does not show any intrinsic directionality, which could affect the crystal symmetry. SAXS measurements showed that CCMV–PAMAM-G6 crystals have a face-centred-cubic (fcc) crystal structure (space group , number 225) with a lattice constant a =40.5 nm ( Fig. 4a–c ). Here the CCMV particles are close-packed—the centre-to-centre distance of CCMV particles is d CCMV–CCMV = a / ✓ 2=28.6 nm, which is ~5% less than in the CCMV–avidin crystal, where a =35.0 nm and d CCMV–CCMV = ✓ 3 a /2=30.3 nm ( Fig. 4a ). A similar CCMV arrangement was recently observed in binary crystals consisting of cationic AuNPs and CCMV that together formed an AB 8 fcc -type structure, which formation was argued to be directed by the location of negative patches on CCMV [20] . In this unit cell, eight AuNPs fill each of the octahedral voids of the fcc-packed CCMV unit cell. The AB 8 fcc structure was directly observed with SAXS and TEM measurements and is illustrated here for comparison ( Fig. 4d ). Owing to the structural similarity between the CCMV–AuNP and CCMV–PAMAM-G6 constituent building blocks and the resulting crystals, we argue that also the CCMV–PAMAM-G6 crystals adopt a similar binary arrangement compared with CCMV–AuNP crystals. Because of the charge distribution geometry on the surface of avidin, the electrostatic potential energy of CCMV–avidin crystal is not minimized by maximal tight packing of the structure as in the case of PAMAM-G6, but rather by the optimal configuration that minimizes the distance between the oppositely charged patches. This leads to an open bcc crystal structure and further to a smaller packing fraction of CCMV particles in the CCMV–avidin crystals. Detailed comparison between the unit cells is presented in Supplementary Table 1 . Modular functionalization of the CCMV–avidin crystals Avidin binds to biotin with high affinity and selectivity ( K d ~10 −15 M) allowing the labelling and modular functionalization of electrostatically assembled CCMV–avidin crystals by uncharged biotin-tagged functional units ( Fig. 5 ). In our study, we verified this by incorporating biotin (5-fluorescein) conjugate ( BF ), biotin-tagged horseradish peroxidase enzyme ( B-HRP ) and biotinylated 5 nm AuNPs ( B-AuNP ) into the crystal structure. The functionalization can be achieved in two ways: by pre-functionalizing avidin with the biotinylated functional unit and then adding the virus particles to form the crystals (Method 1), or by first forming the crystals followed by the addition of biotinylated agent (post-functionalization, Method 2). 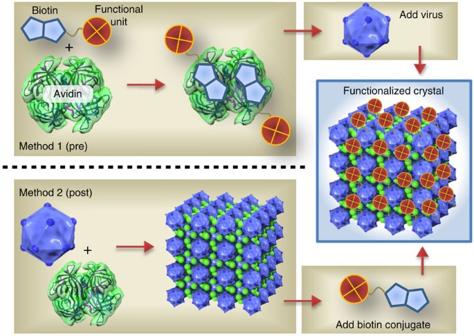Figure 5: Modular pre- and post-functionalization of CCMV–avidin crystals through biotin–avidin interaction. Method 1 and 2 describe the pre- and post-functionalization approaches, respectively. Figure 5: Modular pre- and post-functionalization of CCMV–avidin crystals through biotin–avidin interaction. Method 1 and 2 describe the pre- and post-functionalization approaches, respectively. Full size image Fluorescently labelled crystals carrying BF ( Fig. 6a ) could be efficiently formed by pre- or post-functionalization methods. SAXS curves measured from both samples indicate similar structure as pristine non-functionalized crystals ( Fig. 6b ). BF is very small ( d max ~1.5 nm) compared with the unit cell of the CCMV–avidin crystal and does not affect the structure of the functionalized crystal. BF has a fluorescence emission maximum at λ em ~525 nm ( Fig. 6c ) making the functionalization straightforward to confirm by fluorescence measurements. Crystals were either pre- or post-functionalized in aqueous solution with an amount of BF equivalent to slightly <1 BF molecule per avidin, after which the functionalized crystals were separated from the solution and unbound BF by centrifugation. Both the supernatant (sup. ; 80% of the sample volume) and the sediment (20% of the sample volume) were diluted to the same volume using concentrated NaCl solution to disassemble the crystals and facilitate fluorescence measurements. The integrated fluorescence intensities of pre-functionalized sediment and supernatant were 87% and 16%, respectively, of the pure BF sample fluorescence intensity. For post-functionalized samples, the respective values were 82% and 16% ( Fig. 6d ). This shows that the BF is readily absorbed in the CCMV-lattice regardless of how the BF functionalization is done. 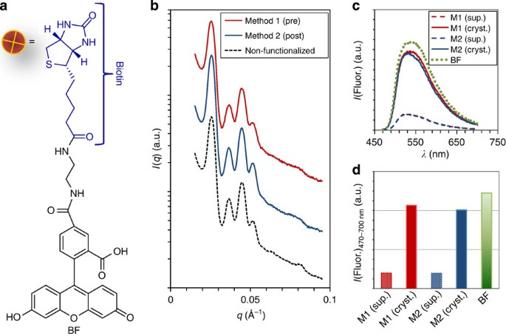Figure 6: Functionalization with fluorescent dyes. Crystals (cryst.) functionalized with (a) biotin (5-fluorescein) (BF) show high degree of crystallinity in SAXS measurements (b) irrespective of preparation method (Methods 1 or 2). Fluorescence spectra (c) and integrated fluorescence intensities (d) show the presence ofBFpredominantly in the crystals but not in the supernatant (sup.). Figure 6: Functionalization with fluorescent dyes. Crystals (cryst.) functionalized with ( a ) biotin (5-fluorescein) ( BF ) show high degree of crystallinity in SAXS measurements ( b ) irrespective of preparation method (Methods 1 or 2). Fluorescence spectra ( c ) and integrated fluorescence intensities ( d ) show the presence of BF predominantly in the crystals but not in the supernatant (sup.). Full size image Crystalline arrays consisting of solely protein-based subunits offer an attractive platform for the creation of novel multifunctional biomaterials. We used B-HRP to functionalize the CCMV–avidin crystals with active enzymes ( Fig. 7a ). HRP catalyses the one-electron oxidation of 3,3′,5,5′-tetramethylbenzidine in the presence of hydrogen peroxide ( Fig. 7b ), which allows straightforward spectrophotometric quantitation ( Supplementary Note 1 ). Structural characterization of crystals pre- or post functionalized with B-HRP shows a bcc crystal structure before and after the enzymatic reaction ( Supplementary Fig. 4 ). Before washing, the functionalized crystals (irrespective of functionalization method) show high enzymatic activity, whereas the separated supernatant shows only low residual activity ( Fig. 7c ; Supplementary Fig. 5 and Supplementary Tables 2 and 3 ). For washed samples, the initial velocity ( V 0 ) for the reaction in the case of functionalized crystals (0.13−0.15 μM s −1 ) is ~2 orders of magnitude higher compared with the residual-free enzymes in the solution (~0.007 μM s −1 ; Fig. 7d ), demonstrating that active enzymes can be efficiently loaded to and concentrated by the crystalline assemblies. 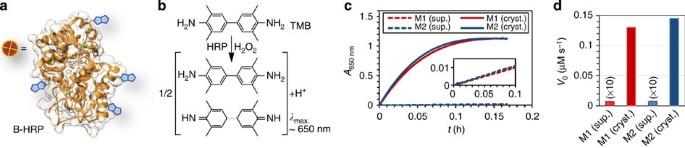Figure 7: Functionalization with enzymes. Biotinylated horseradish peroxidase (B-HRP,a) catalyses the one-electron oxidation of 3,3',5,5'-tetramethylbenzidine (TMB) to a blue-coloured charge transfer complex (b). Progress curves (c) and the derived initial velocities (V0,d) show that the crystals have a high catalytic activity (V0>0.1 μM s−1) after functionalization. Figure 7: Functionalization with enzymes. Biotinylated horseradish peroxidase ( B-HRP , a ) catalyses the one-electron oxidation of 3,3',5,5'-tetramethylbenzidine (TMB) to a blue-coloured charge transfer complex ( b ). Progress curves ( c ) and the derived initial velocities ( V 0 , d ) show that the crystals have a high catalytic activity ( V 0 >0.1 μM s −1 ) after functionalization. Full size image Furthermore, we compared the enzyme activity in samples with different structure morphologies and showed that only the crystalline samples could be efficiently separated or concentrated while maintaining high enzyme activity. These features were not possible to achieve with separated and concentrated amorphous structures, as they lose their enzyme activity due to uncontrolled aggregation. Free-avidin– B-HRP complexes in comparison do not allow concentrating the samples. Particularly, the crystalline complexes allow the packing of enzymes in controlled manner to a minimal volume, which allows high catalytic activity to be maintained ( Supplementary Fig. 6 , Supplementary Table 4 and Supplementary Note 2 ). To investigate the incorporation of plasmonic nanoparticles into the protein crystals, biotin-tagged AuNPs ( B-AuNP s) with a metal core diameter of ~5 nm were used ( Fig. 8a ). Scattering curves obtained from B-AuNP pre-functionalized crystals shows clearly the presence of bcc lattice and B-AuNP form factor P (q), which dominates the scattering due to the high electron density of gold. Taking the B-AuNP P (q) into account, the measured scattering curve is in excellent agreement with the scattering patterns from non-functionalized samples and comparable to crystals functionalized with B-HRP or BF ( Supplementary Fig. 7 ). However, the Bragg reflections are not enhanced, which implies that the B-AuNP s are heterogeneously distributed in the crystals ( Fig. 8b ). TEM images of AuNP-functionalized crystals further support heterogeneous distribution and show that the AuNPs are well-dispersed throughout the CCMV–avidin crystal and do not occupy defined lattice points ( Fig. 8c ). Also the observed redshift in the absorption maximum for gold particles indicates that they are in close proximity ( Supplementary Fig. 8 and Supplementary Note 3 ). Yet, the organization of the particles is clearly directed by the crystal and tightly clustered particles are absent. TEM images comparing clustered and crystal-dispersed AuNPs reveal a clear difference ( Fig. 8d ). In comparison, we have previously shown that cationic AuNPs can electrostatically self-assemble with CCMV particles to produce AB 8 fcc -type binary superlattices, where the AuNPs occupy the octahedral voids of close-packed CCMV-lattice with an fcc structure [20] . TEM image viewing such a lattice along the [110] projection axis is shown in Fig. 8e . Image Fourier transform and inverse Fourier transform calculated with selected Fourier components indicate high degree of order ( Fig. 8f ). 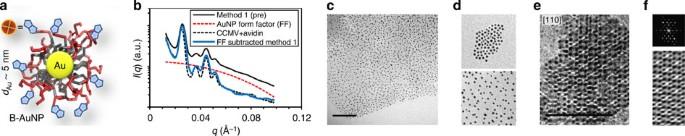Figure 8: Functionalization with AuNPs. Biotinylated gold nanoparticles (B-AuNPs) with a gold core diameter of ~5 nm (a) can be incorporated to crystals according to the measured SAXS curves. Form factorP(q) of the AuNPs dominates the scattering pattern indicating heterogeneous distribution of AuNPs in the crystal (b), which can also be visualized with TEM (c). Scale bar, 150 nm. (d) An AuNP cluster in the absence of protein crystals compared with a magnified view of the AuNP-functionalized crystals. Dimensions for the images are 150 × 150 nm. A comparison to a previously obtained AB8fcc-type CCMV–AuNP binary crystals viewed along the [110] projection axis (e). Here the AuNPs occupy defined lattice points. (f) Fourier transform from imageeand inverse Fourier transform calculated with selected Fourier components. Figure 8: Functionalization with AuNPs. Biotinylated gold nanoparticles ( B-AuNP s) with a gold core diameter of ~5 nm ( a ) can be incorporated to crystals according to the measured SAXS curves. Form factor P (q) of the AuNPs dominates the scattering pattern indicating heterogeneous distribution of AuNPs in the crystal ( b ), which can also be visualized with TEM ( c ). Scale bar, 150 nm. ( d ) An AuNP cluster in the absence of protein crystals compared with a magnified view of the AuNP-functionalized crystals. Dimensions for the images are 150 × 150 nm. A comparison to a previously obtained AB 8 fcc -type CCMV–AuNP binary crystals viewed along the [110] projection axis ( e ). Here the AuNPs occupy defined lattice points. ( f ) Fourier transform from image e and inverse Fourier transform calculated with selected Fourier components. Full size image In summary, we have shown the electrostatic self-assembly of native biological building blocks into ordered binary lattices, which allow the intrinsic biofunctionality of proteins to be used. The charge and size ratio of the particles have a significant role in the lattice formation: avidin is large enough to function as a spacer between CCMV particles and also the geometry of the patches on avidin can direct the lattice formation. In this, our method resembles Nature’s approach to pack virus particles with crystalline polyhedrin proteins [51] . Furthermore, we have demonstrated that the CCMV–avidin crystal can be functionalized in a modular and straightforward manner by using biotin-tagged functional units from different classes of the nano-sized building blocks [52] . We emphasize that the method is not limited to the produced examples of small molecules, enzymes and plasmonic particles, but can be broadly applied with various different biotin tags. This approach, where a third component is added to a binary crystal, mimics the process of topotactic intercalation [15] , and demonstrates its use with macromolecules in biologically relevant environment, thus paving way for the successful design and preparation of complex protein assemblies found in nature [53] . Materials CCMV was produced and isolated from California black-eye peas ( Vigna unguiculata ). Lyophilized avidin from egg white, PAMAM-G6, poly(acrylic acid) and biotin (5-fluorescein) conjugate were supplied by Sigma-Aldrich. Avidin was dissolved in Milli-Q water (10 mg ml −1 ), and biotin (5-fluorescein) conjugate was dissolved in dimethyl sulfoxide (10 mg ml −1 ). Biotin HRP was supplied by Life Technologies, and biotinylated AuNPs with 5 and 15 nm gold core were supplied by Cytodiagnostics ( Supplementary Note 4 ). Dynamic light scattering DLS equipment (Zetasizer Nano Series, Malvern Instruments) equipped with a 4-mW He–Ne ion laser at a wavelength of 633 nm and an Avalanche photodiode detector at an angle of 173° was used to measure both the hydrodynamic diameter and the electrophoretic mobility. Experiments were carried out at 25 °C and before the sample preparation, CCMV and avidin solution were filtered (Acrodisc GHP 0.45 μm filter and Acrodisc GHP 5 μm filter, respectively). For titration series, the initial sample contained CCMV as an aqueous solution (0.03 mg ml −1 ) to which avidin solution (0.03 mg ml −1 ) was sequentially added until mass ratio m (CCMV) : m (avidin) of 1: 0.75 was reached. Samples were thoroughly mixed after each avidin addition. The electrophoretic mobility was measured from five different samples that consisted of CCMV (0.05 mg ml −1 ), to which avidin (1 mg ml −1 ) was added to reach mass ratios m (CCMV) : m (avidin) of 1:0, 1:0.04, 1:0.16, 1:0.32 and 1:0.75. The measurements were carried out in Plastibrand semi-micro poly(methyl methacrylate) cuvettes. Zetasizer software (Malvern Instruments) was used to obtain the scattering intensity (count rate), particle size distributions and the electrophoretic mobility. DLS data were not further treated, except for the normalization of the count rate in Fig. 2c by multiplying with a normalization constant C v to compensate for the dilution of the sample during the titration ( C v =volume/initial volume). Small-angle X-ray scattering The samples were prepared by adding 1.25 μl NaCl water solution in 5 μl CCMV solution (10 mg ml −1 ) to adjust the ionic strength after which 3.75 μl avidin (10 mg ml −1 ) was added under stirring. In biotin (5-fluorescein), biotin AuNP and biotin HRP-functionalized samples, the functional unit was added either to the avidin water solution before the addition of avidin (pre-functionalization) or to the premade CCMV–avidin crystals (post functionalization). The liquid samples were sealed between two Kapton foils during the SAXS measurements, and the sample environment was evacuated to reduce scattering from air. The SAXS was measured using a rotating anode Bruker Microstar microfocus X-ray source (Cu K α radiation, λ =1.54 Å). The beam was monochromated and focused by a Montel multilayer focusing monochromator (Incoatec). The X-ray beam was further collimated by a set of four slits (JJ X-ray) resulting in the final spot size of <1 mm at the sample position. The scattered intensity was collected using a Hi-Star 2D area detector (Bruker). Sample-to-detector distance was 1.59 m, and silver behenate standard sample was used for calibration of the length of the scattering vector q . One-dimensional SAXS data were obtained by azimuthally averaging the 2D scattering data. The magnitude of the scattering vector q is given by q =4 π sin θ / λ , where 2 θ is the scattering angle. Details of data analysis are presented in Supplementary Methods . TEM imaging CCMV–avidin sample (15 mM NaCl) was prepared in the same way as for SAXS measurements and diluted 1: 9 with 15 mM NaCl. The sample was vitrified on a TEM grid and imaged at liquid nitrogen temperature. Vitrification was done using FEI Vitrobot Mk3 in a saturated water vapour environment. Sample volumes of 3 μl were placed on Quantifoil R 3.5/1 grids and the excess sample was blotted away with filter paper. Blot time and drain time were both 1 s. After blotting, the grids were plunged into liquid ethane/propane (1:1) solution that was cooled with liquid nitrogen surrounding the ethane/propane vessel. Vitrified samples were cryo-transferred to the microscope. Imaging was performed with JEOL JEM-3200FSC equipment operating at a 300-kV accelerating voltage and specimen temperature of ~86 K. Conventional TEM imaging of CCMV–avidin crystals functionalized with 5 nm AuNPs was carried out with Tecnai 12 Bio-Twin transmission electron microscope (FEI) using an acceleration voltage of 120 kV. The sample was added on Quantifoil R 3.5/1 grid and the excess sample was blotted away with filter paper. The functionalized CCMV–avidin–AuNP samples were imaged both with and without uranyl acetate (negative) staining. Spectroscopy Ultraviolet (UV)-visible spectra and enzyme progress curves were measured using PerkinElmer LAMBDA 950 UV/Vis spectrophotometer. Fluorescence spectra were recorded using a QuantaMaster 40 spectrofluorometer from Photon Technology International. A double-excitation monochromator was used in the measurements to decrease the stray light level, and the slits in excitation and emission monochromators were set to 5 nm. Fluorescence spectra were recorded using standard 90° measurement geometry without excitation or emission filters. Excitation and followed emission wavelength range were 460 and 470–700 nm, respectively. The fluorescence spectra were corrected by using instrument’s excitation and emission corrections provided by the manufacturer. Fluorescence spectra were recorded in high-quality quartz cells with a 3-mm path length. The pre- and post-functionalized crystals were prepared in the same way as the BF SAXS samples. The functionalized samples were diluted into a volume of 100 μl and centrifuged. The samples were then divided into 80 μl of supernatant and 20 μl of sediment to which NaCl solution was added to get a final volume of 100 μl and NaCl concentration of 100 mM, a concentration that makes the functionalized lattices disintegrate. This process was necessary in order to reduce scattering from large crystals. A reference sample was prepared with the same total amount of BF . How to cite this article: Liljeström, V. et al. Self-assembly and modular functionalization of three-dimensional crystals from oppositely charged proteins. Nat. Commun. 5:4445 doi: 10.1038/ncomms5445 (2014).